Focusing light with a flame lens The lens is a well-understood optical component used for focusing light, but is almost exclusively made in the solid-state form and, thus, suffers from optical damage at high powers. Attempts to overcome this through the use of non-solid graded-index media for lensing, for example, heated gasses, have found limited application owing to their long focal lengths. Here we describe the first flame lens, which produces a sharp focus with very little stray light and has a fourfold increase in focal power per unit length over previous gas lenses. Such gas devices remain topical due to their inherent ability to deliver high-power laser beams: our flame lens has a ‘damage’ threshold that is several orders of magnitude higher than that of most conventional lenses and is immediately repaired after damage for reuse, and thus will be of use in focusing high-irradiance laser beams. Gas lenses—using air to focus light—were invented several decades ago [1] , [2] , [3] , [4] and later applied in a range of demonstrations, including laser drilling [5] , the generation of plasmas [6] and telescopy [7] . All gas lenses rely on the production of a refractive index gradient to focus or defocus natural or laser light propagating through the lens, usually along some axis of symmetry. The gradient can be generated either by heating the walls of a long tube [1] , [2] or by colliding shock waves in air [8] . Further control and stabilization of the gradient can be maintained by rotation, as in the spinning pipe gas lens [5] , [9] . Unfortunately, such devices have suffered from intrinsic aperture limitations; they are cumbersome and they require complex power supplies or moving parts, and have been optically weak owing to their low refractive index gradients. There has also been interest in the optics of flames [10] , where the passive optical properties of flames have long been used in spectroscopy [10] , [11] , [12] , [13] , and flames have been used to line-focus laser light [14] , [15] , [16] . Optical devices based on gases and flames have the advantage of a high damage threshold. Although conventional lenses are susceptible to optical damage, a known limitation in advancement of high-power laser systems in the petawatt regimes and beyond, gases and plasmas have very high breakdown thresholds [17] of the order of 10 13 W cm −2 and 10 17 W cm −2 , respectively, and thus flames offer several orders of magnitude increase in damage threshold over conventional solid-state optical components, which damages at levels of 10 9 W cm −2 for coated elements and 10 12 W cm −2 for polished substrates [18] , [19] . To date, no studies have taken this concept further to create high damage threshold lens. In this study we outline the concept of a flame lens, demonstrate it experimentally and perform a full computational fluid dynamics (CFDs) model to validate the concept theoretically. We demonstrate the efficacy of the lens in two proof-of-principle experiments: the first verifying the ability to image a highly chromatic object and the second illustrating the focal quality of the lens in creating circular holes laser-drilled in plastic targets. We show that our flame lens produces a sharp focus by gas lens standards and is four times stronger per lens unit length than a conventional gas lens. Unlike previous gas lens devices, the flame lens has no moving parts or electrical circuits, nor does it suffer from aperture restrictions. The composite flame lens Our composite flame lens ( Fig. 1 ) consists of a short (5 cm) tubular gas lens ( Fig. 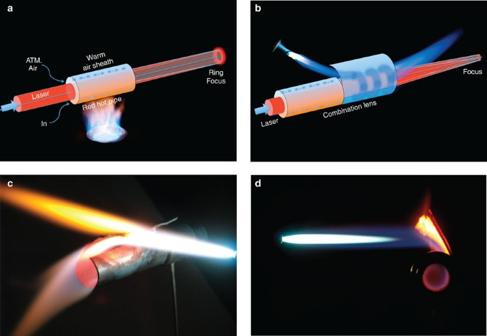Figure 1: Concept and experimental realization of the flame lens. (a) Schematic of the ring focus formed by a gas lens. (b) Schematic of the flame lens with a vortex flame to produce sharp focusing. (c) A pencil flame from an oxyacetylene burner is injected into the tube. (d) The vortex nature of the flame forms a luminous sheath near the tube wall. 1a ) with an aperture of 10 mm, followed by a spiral flame lens ( Fig 1b ) of length 2.5 cm. The stainless steel of both lenses is heated to ~400 °C (almost ‘red hot’). The drawn air tubular lens is a conventional hot air lens, which works by aspiring cold atmospheric air down the tube. It is known [5] that such lenses must have an aperture of less than 7 mm, a radial temperature difference of less than 100 °C and a length between 30 cm and 1 m. A short, large aperture lens only refracts the outer rays to produce a ring focus; so this drawn air lens would not point-focus on its own. We introduce a second lens, the spiral flame lens, which acts mainly on the inner rays to form the composite lens ( Fig. 1b ). In the spiral or vortex flame lens, a single oxyacetylene or propane pencil flame is injected into an 11-mm diameter cylinder, so that it spirals along the 2.5-cm long flame tube ( Fig. 1c ), generating a visible luminous cylindrical sheath ( Fig 1d ). This sheath establishes the required refractive index gradient for lensing. Evidently, the very high temperature of the flame creates a much steeper temperature and refractive index gradient than in a conventional gas lens. However, as will be shown later, there is significant stray light around the focal spot as well as a ring of non-refracted peripheral light. By adding the tubular lens to the spiral flame lens so that the two fit tightly together ( Fig. 1b ), it is possible to eliminate both the stray light and the unfocused ring. Figure 1: Concept and experimental realization of the flame lens. ( a ) Schematic of the ring focus formed by a gas lens. ( b ) Schematic of the flame lens with a vortex flame to produce sharp focusing. ( c ) A pencil flame from an oxyacetylene burner is injected into the tube. ( d ) The vortex nature of the flame forms a luminous sheath near the tube wall. Full size image To understand the composite flame lens, one turns to conventional gas lens theory [1] , [2] , [3] and earlier flat flame experiments [16] , where the lens is modelled as a graded index medium established through the temperature (density) gradient transverse to the propagation. The refractive index, n , as a function of temperature, T , is taken to obey the Gladstone–Dale law for air [20] , so that the change in refractive index between hot air at the wall temperature ( T = T w ) and standard temperature and pressure (STP) air at the edge of the sheath ( T = T 0 ) is given by One assumes from previous studies [21] , [22] that the heated tube generates a parabolic average refractive index profile as a function of lens radial position, r , so that where γ is a constant determined from the lens properties (see later). To estimate the focal length of such a medium, consider the phase-only transmission function for a light ray passing through the flame lens of effective length l eff , expressed as where k =2 π / λ and λ is the wavelength of the light. Comparing equation (4) with the well-known transmission function for a thin lens of focal length f , t =exp[– ikr 2 /2 f ], we find a pragmatic formula for the focal length of the flame lens where l eff is the effective length of the lens. We start by considering the tubular lens and the spiral flame lens as separate optical elements. Experiments and simulations show that the tubular gradient only extends about 2 or 3 mm from the wall. Weak gradient refraction [20] predicts a refraction angle of , where Δr is the thickness of the warm air sheath and l eff is the effective length of the lens, which is a parameter of order half the actual length and which depends on the air flow (in conventional gas lenses the effective length is the actual length reduced by the distance needed to establish a gradient [21] , [22] ). For our experimental conditions ( T w ~400 °C, Δr ~3 mm and l eff ~2.5 cm), the divergence of the rays is θ~ 1 mrad. For rays starting at r =4 mm, the radial displacement after 2.5 m is ~3 mm. We thus see that the flame lens need hardly refract these rays for them to arrive nonetheless in the focal region. This general behaviour of the drawn air tubular lens has been confirmed by running a preheated flame lens on pure oxygen and no flame. For the spiral flame lens we make the following assumptions. First, the temperature coefficient ( T w − T 0 )/ T w ≈0.8, as the wall temperature is now the flame temperature and is very high ( T w ≈1300 K). Second, from simulations and experiments we know that the effective tube radius is reduced to about 3.5 mm to take the existence of the non-refracting peripheral flame into account (see, for example, the dark core of the flame lens in Fig. 1d ). And lastly, the effective length is half of the 2.5-cm real length, because the pitch of the flame spiral is at 45 °, reducing its refractive effects. With these assumptions we find f ≈2 m, a four times increase in focal power per unit length over conventional gas lenses. Computational model A CFD model of the lens was developed to allow predictions of the density and temperature of the air in the flame lens as a function of axial and radial position, and time. We modelled a stainless steel lens housing of length 75 mm (50 mm for the tubular lens component and 25 mm for the flame lens component), and with inner and outer diameters of 10 mm and 11 mm, respectively. The model consisted of two phases: a fluid phase (air—represented with 274,682 computational cells) and a solid phase (carbon steel—represented with 79,323 computational cells). The pressure and density of the air were allowed to change in accordance with the ideal gas law, and the temperature of the steel was allowed to change through the process of conjugate heat transfer. The calculated density, temperature and gas velocity distributions are shown in Fig. 2 for four cross-sectional positions in the flame lens. The physical structure of the lens is shown as a light grey outline. Near the centre of the lens, the density and temperature (and, hence, refractive index) variation is approximately symmetric, but changes over the length of the lens due to the nature of the vortex flame. In Fig. 3 we show the density, temperature and gas velocity a few seconds after the flame is injected in the lens. The temperature cross-section along the length of the flame lens shows that near the exit of the pipe the temperature distribution is rather complicated and not symmetric about the beam axis, which is parallel to the pipe walls. This accounts for the majority of the aberrations introduced to the laser beam. 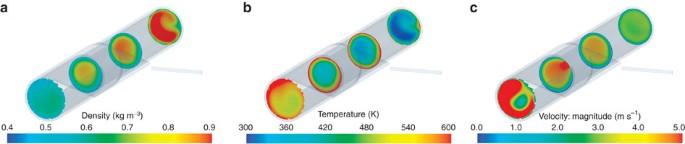Figure 2: CFD model results of the flame lens at four axial positions. (a) False colour plot of the CFD calculated density at the two ends of the lens and at two central regions. The same is shown for (b) temperature and (c) gas velocity. Near the centre of the lens the cross-sectional profiles have approximate radial symmetry. The flame lens structure is shown in grey together with the injection nozzle of the flame (grey rod). Figure 2: CFD model results of the flame lens at four axial positions. ( a ) False colour plot of the CFD calculated density at the two ends of the lens and at two central regions. The same is shown for ( b ) temperature and ( c ) gas velocity. Near the centre of the lens the cross-sectional profiles have approximate radial symmetry. The flame lens structure is shown in grey together with the injection nozzle of the flame (grey rod). 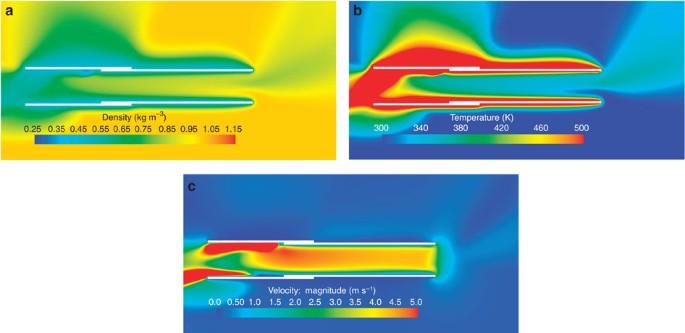Figure 3: CFD model results of the flame lens along its length. (a) False colour plot of the CFD calculated density cross-section along the length of the lens, shown a few seconds after the flame is injected. The same is shown for (b) temperature and (c) gas velocity. The flame lens structure is shown in white. Full size image Figure 3: CFD model results of the flame lens along its length. ( a ) False colour plot of the CFD calculated density cross-section along the length of the lens, shown a few seconds after the flame is injected. The same is shown for ( b ) temperature and ( c ) gas velocity. The flame lens structure is shown in white. Full size image By considering the cumulative optical path length through the lens, the effective phase change experienced by an optical beam can be calculated from equation (4). Such a profile is shown in Fig. 4a , and as a refractive index cross-section in Fig. 4b . 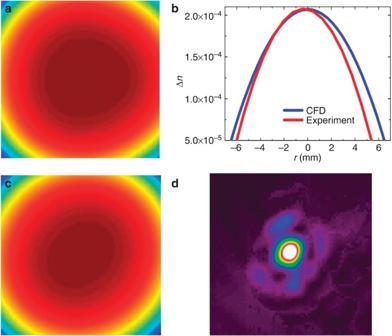Figure 4: CFD and experimental data. (a) False colour plot of the CFD calculated cumulative phase change due to the flame lens, in waves from 0 (red) to −2.5 (dark blue). The scale bar is 1 mm. (b) Inferred refractive index profiles from the CFD and experimental data. (c) False colour plot of the experimentally measured cumulative phase change due to the flame lens, in waves from 0 (red) to −2.5 (dark blue). (d) Measured irradiance profile of the focal spot of the flame lens. Figure 4: CFD and experimental data. ( a ) False colour plot of the CFD calculated cumulative phase change due to the flame lens, in waves from 0 (red) to −2.5 (dark blue). The scale bar is 1 mm. ( b ) Inferred refractive index profiles from the CFD and experimental data. ( c ) False colour plot of the experimentally measured cumulative phase change due to the flame lens, in waves from 0 (red) to −2.5 (dark blue). ( d ) Measured irradiance profile of the focal spot of the flame lens. Full size image Although the phase profile shown in Fig. 4a have higher-order aberrations, the predominant contribution is defocused, giving rise to the approximately parabolic refractive index profile as shown in Fig. 4b . Flame lens performance Experimental results confirm the concept and theoretical analysis. A Helium–Neon laser beam was transmitted through the flame lens and it formed a visual point focus at a distance of about 2.5 m, in good agreement with the predicted value of ~2 m. The focal spot had a central peak of radius w =0.46±0.06 mm only a few times diffraction limited ( Fig. 4d ). A movie of the changing focal spot due to imperfections in the entry angle of the flame is shown in Supplementary Movie 1 . The measured phase of the laser beam on exiting the flame lens was used to compute the cumulative phase change due to the lens ( Fig. 4c ) and the experimentally inferred refractive index gradient ( Fig. 4b ). The refractive index profiles of the CFD and experimental data match well, with parabolic coefficients (from equation (3)) given by γ 2 =3.6 × 10 –6 mm –2 and by γ 2 =3.2 × 10 –6 mm –2 , respectively. From the experimental data, the focal length of the lens was inferred (equation (5)) to be f =2.4±0.5 m, corroborating the aforementioned analysis, whereas the focal length as calculated from the CFD data was found to be f =2.2 m. There is good quantitative agreement between the CFD model predictions and the experimental data; it is expected that the agreement would improve if the initial conditions of the flame were known more precisely, for example, the precise injection angle, velocity and temperature of the flame. Two high-power focusing experiments were performed to demonstrate the ability of the lens to withstand high peak powers. In the first experiment, a pulsed Nd:YAG laser was used to successfully drill a hole in a plastic target ( Fig. 5 ). With the flame turned off, the laser beam makes a barely perceptible sound as each unfocused pulse illuminates the plastic. The moment the flame is ignited loud ‘cracks’ are audible and a bright plasma plume appears. Varying the flame intensity and its entry level into the lens changes its strength. Such varifocal behaviour may be useful in, for example, maintaining a focus on a moving target or machining high aspect ratio materials. In the second experiment, a high-irradiance Ti:Sapphire laser pulse was focused using the flame lens. The initial expanded spot entering the lens had a peak irradiance of ~10 10 W cm −2 and could be increased to ~10 16 W cm −2 by prior focusing. An important aspect of the flame lens is its ability to withstand high laser intensities. The laser spot was focused into the flame lens and the breakdown threshold recorded both for the air and the flame regions. Breakdown was observed for values of the order of ~10 13 W cm −2 for both; when the same spot was focused into the hottest and most intense part of the flame, no breakdown was observed even at significantly higher peak intensities. 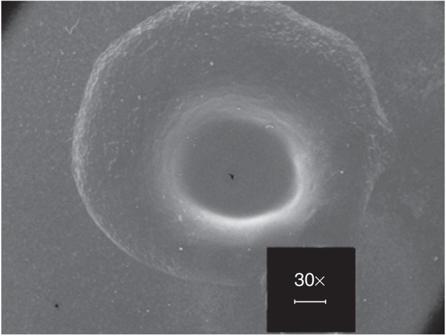Figure 5: Flame lens focusing. A hole drilled in plastic with a nanosecond pulsed laser. The scale bar is 400 μm. Figure 5: Flame lens focusing. A hole drilled in plastic with a nanosecond pulsed laser. The scale bar is 400 μm. Full size image Finally, a proof of principle experiment demonstrated the imaging properties of the flame lens. We present here the first image by a flame lens. 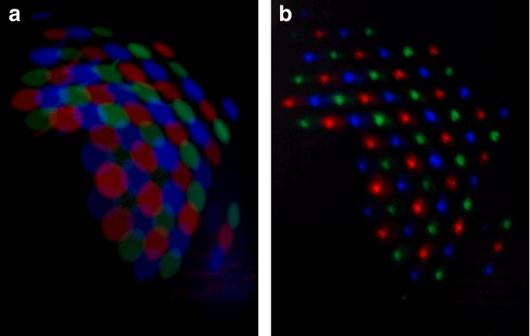Figure 6: Flame lens imaging of multicoloured LEDs. (a) Image with the flame turned off (no lens). (b) Image with the flame turned on. Figure 6a shows the illumination due to some seventy light-emitting diodes (LEDs) forming a blurry image of Africa through the switched-off flame lens. When the lens was ignited, an in-focus picture of the object was formed ( Fig 6b ). A notable point is that all the LEDs are focused in the same degree, corresponding to a field of view of some 70 mrad, or over 3°. Figure 6: Flame lens imaging of multicoloured LEDs. ( a ) Image with the flame turned off (no lens). ( b ) Image with the flame turned on. Full size image Another way of explaining why the combination flame lens is a considerable improvement on either a hot-drawn air lens or a spiral flame lens comes from comparison with other gas and flame experiments. The important point is that the central part of any flame is a poor refractor. Previous experiments [16] in which pencil beams were made to traverse a flat flame showed that the strongest refraction occurs at the flame front, followed by weakening refraction, as the pencil beam moves out of the flame’s luminous sheath. This explains why only the light traversing the central regions of the spiral flame lens is refracted and not the peripheral. The second way of explaining the spiral flame’s behaviour is to consider the spiral flame as a curved version of the flat flames. The gradually decreasing refraction with increasing distance from the flame (that is, decreasing flame lens radius) focuses laser light exactly as in a converging solid-state lens. An interesting experimental observation is that the composite lens also works well at strong inclination, for example, at 45 °. Once heated, one may even dispense with the flame: convection currents maintain the focusing for several minutes until the metal cools. This is because a heated inclined tube (with no gas injection) generates the same funnel as found in the horizontal version. One of the key motivations for considering such lenses is their high damage threshold. Our results are consistent with reported values of gas and plasma breakdown, which indicate that the flame lens would have a damage threshold approximately three orders of magnitude higher than conventional coated optics [17] . Indeed, a proposal to circumvent optical damage in high-irradiance amplifying systems has recently been mooted: to replace metre-scale beams with millimetre-diameter plasmas through Raman amplification [23] . Laser damage in solid-state optics is of course permanent, and in many cases when the optics are not damaged the time frame for the cooling of the optics can run into hours. In contrast, should the damage threshold in the flame lens be exceeded, the lens recovers from this in microsecond time scales—virtually instantaneously in the context of most high-power laser experiments. A present disadvantage of the flame lens is the relatively high aberrations, as noted from the distorted focused beam in Fig. 4d and quantified in Fig. 7 . The CFD model predicts cones of cold, as well as exiting plumes of hot air from the flame lens. The cones are obvious focusing elements—albeit imperfect—as they are far from parabolic, whereas the plumes account for further aberration (described in Fig. 7 as Zernike aberrations). This suggests a route to improving the optical performance of the lens, through aerodynamically engineering the lens structure to minimize the impact of the exit plume on the propagating light, for example, by diverting the flume away from the optical path. 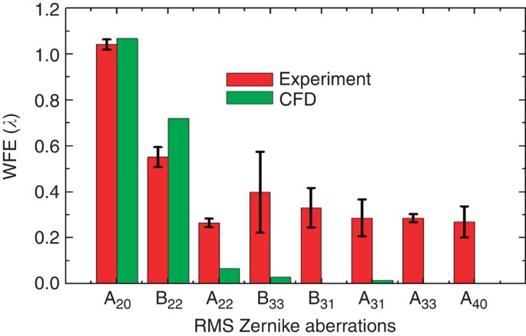Figure 7: Measured and simulated wavefront error. The simulated (CFD) wavefront error (WFE) considers only the root mean square (RMS) aberrations introduced within the length of the flame lens, whereas the measured data includes both this and the additional aberrations due to the path outside the flame lens. The high-order aberrations are due to the exit plumes. The error bars depict the s.d. Figure 7: Measured and simulated wavefront error. The simulated (CFD) wavefront error (WFE) considers only the root mean square (RMS) aberrations introduced within the length of the flame lens, whereas the measured data includes both this and the additional aberrations due to the path outside the flame lens. The high-order aberrations are due to the exit plumes. The error bars depict the s.d. Full size image In conclusion, we have demonstrated a novel method of employing flames to make a virtually damage-free lens for high-power laser applications. It is possible to progress from this first proof-of-concept flame lens to larger aperture or shorter focal length devices of higher optical quality, for example, by increasing the length and operating at higher pressures. Petawatt lasers are demonstrating potential applications in, for example, medicine and fast ignition of fusion targets, but on a single pulse basis. Repetitively, pulsed petawatt lasers will present damage challenges for conventional optics, but not for a flame lens. The flame lens has none of the aforementioned disadvantages of conventional optics, is inexpensive and is a major improvement on all previous gas lens designs—it has no moving parts, no electrical contacts and shows a fourfold performance improvement. This bodes well for the flame lens as a future technology if the present prototype is carefully re-engineered for optical quality. Laser experiments A Helium–Neon laser (Thor Labs) was used for the low-power experiments and the focal spot recorded with a CCD camera (Spiricon Inc.). The drilling experiment was performed with a Q-switched Nd:YAG laser (Spectra Physics) and was operated at ~300 mJ per pulse, with a pulse length (full width at half maximum) of 20 ns. The high-irradiance damage and focusing test was done with a mode-locked Ti:Sapphire laser (Clark MXR), amplified to pulse energies of up to 1 mJ at a repetition rate of 1,000 Hz, with a pulse width (full width at half maximum) of 150 fs at a wavelength of 775 nm. Aberration measurement We used the Zernike basis for describing optical aberrations, in which a set of Zernike polynomials is defined on a unit circle, with the magnitude of the weighting coefficients signifying how much each aberration contributes to the overall wavefront variance [24] , [25] . We made use of the laser beam quality factor, M 2 , as our measurable, as it is invariant for propagation through an aberration-free system, but increases with optical aberrations other than piston, tilt and defocus [26] . This allowed us to separate the lensing action from the impact of aberrations. In our experiments a beam from a Helium–Neon laser was expanded to a 3.28 mm 1/ e 2 radius beam, attenuated through neutral density filters, and then steered into the flame lens. The wavefront of the exit beam was measured with a Shack–Hartmann wavefront sensor (Wavefront Sciences, model CLAS 2D), with a 69 × 69 lenslet array, placed 91 cm from the exit face of the tube to protect the sensor from heat damage. A reference wavefront (with no flame lensing) was subtracted from all further wavefront measurements. The experiment was repeated 24 times to gather lensing statistics and to test repeatability. A Zernike aperture radius of 3.41 mm was applied throughout the experiment. Numerical simulations The flame lens was modelled using commercial CFD code (StarCCM+) to solve the Reynolds-averaged Navier–Stokes equations numerically, using a finite volume approach. This approach required the generation of a mesh representing the physical domain to enable the conversion of the partial differential Navier–Stokes equations to a set of algebraic equations. The mesh consisted predominantly of hexahedral elements, although a limited number of polyhedral cells were used to ensure that the physical domain was accurately represented. Local grid refinement was done in areas where high gradient in the flow variables were expected, for example, near the tube and directly above it. We modelled a lens of length 75 mm and with inner and outer diameters of 10 mm and 11 mm, respectively. The model consisted of two phases: a fluid phase (air—represented with 274,682 computational cells) and a solid phase (carbon steel—represented with 79,323 computational cells). The pressure and density of the air were allowed to change in accordance with the ideal gas law and the temperature of the steel was allowed to change through the process of conjugate heat transfer. Initially, the air was at rest at STP conditions. It was assumed that the injected flame had an initial temperature of 2,696 °C and a velocity of 330 ms –1 . Turbulence was modelled using the k-epsilon turbulence model with wall functions. The steel was initially at 400 °C. The simulations modelled a total period of 5 s. How to cite this article: Michaelis M. M., et al . Focusing light with a flame lens. Nat. Commun. 4:1869 doi: 10.1038/ncomms2894 (2013).